Length regulation of mechanosensitive stereocilia depends on very slow actin dynamics and filament-severing proteins Auditory sensory hair cells depend on stereocilia with precisely regulated lengths to detect sound. Since stereocilia are primarily composed of crosslinked, parallel actin filaments, regulated actin dynamics are essential for controlling stereocilia length. Here we assessed stereocilia actin turnover by monitoring incorporation of inducibly expressed β-actin-GFP in adult mouse hair cells in vivo and by directly measuring β-actin-GFP turnover in explants. Stereocilia actin incorporation is remarkably slow and restricted to filament barbed ends in a small tip compartment, with minimal accumulation in the rest of the actin core. Shorter rows of stereocilia, which have mechanically gated ion channels, show more variable actin turnover than the tallest stereocilia, which lack channels. Finally, the proteins ADF and AIP1, which both mediate actin filament severing, contribute to stereocilia length maintenance. Altogether, the data support a model whereby stereocilia actin cores are largely static, with dynamic regulation at the tips to maintain a critical length. Auditory and vestibular hair cells are specialized sensory cells in the inner ear that depolarize in response to mechanical force. This function depends on a specialized cellular architecture that features a precisely structured bundle of actin-based protrusions on the apical surface of the cell called stereocilia. Auditory hair cell bundles have three rows of stereocilia of decreasing height, where row 1 is the tallest row and rows 2 and 3 are successively shorter. Within a row, stereocilia are very similar in height. The tips of stereocilia in the shorter rows are connected to the sides of the adjacent taller row by tip links, which are composed of cadherin-23 and protocadherin-15 heteromers [1] . Mechanosensitive ion channels in the shorter row stereocilia are coupled to tip links, and deflections of the bundle transfer tension through tip links to open mechanotransduction channels [2] , [3] , [4] . Maintaining precisely registered stereocilia heights within rows results in uniform tension on all of the tip links in the bundle and synchronous gating of mechanotransduction channels. Importantly, mammalian hair cells are not replaced if they die, so maintenance of stereocilia architecture throughout life is required for continued auditory function. Stereocilia are cytoskeletal structures primarily formed from actin filaments organized into a paracrystalline array by various crosslinking proteins [5] . The barbed ends of the actin filaments, which have a higher affinity for actin monomers than the pointed ends, are uniformly oriented towards the stereocilia tip [6] . Unlike related cellular structures such as microvilli, which rapidly turn over bundled arrays of F-actin by treadmilling [7] , our recent data instead support a model positing that the F-actin cores of stereocilia are remarkably stable with exceptionally slow turnover of actin filaments [8] . In that study, multi-isotope imaging mass spectrometry and conditional ablation of actin isoforms each suggested that actin in a small ( ∼ 0.5 μm) region at stereocilia tips is dynamic, whereas actin filaments constituting the remainder of the stereocilia core are replaced slowly over a timecourse of several months [8] . The mechanisms that regulate the extreme stability of actin in the stereocilia core and the more dynamic turnover at stereocilia tips are unknown. However, the stereocilia proteome includes numerous actin-binding proteins that potentially influence actin behaviour [9] . Actin crosslinkers and barbed end capping proteins are expressed at high levels and likely affect filament stability. Proteins that destabilize actin are also present, including AIP1 and actin depolymerizing factor (ADF) [9] . AIP1 (also called WDR1) synergizes with cofilin to accelerate actin severing and disassembly [10] , [11] , [12] , [13] , [14] while also cooperating with capping protein to regulate filament barbed ends [15] , [16] . ADF (also called destrin), is a well-known actin-severing protein that is functionally and structurally similar to cofilin [17] . These proteins induce breaks in actin filaments and can stimulate actin assembly or disassembly depending on the cellular conditions [18] , [19] , [20] . Severing activity is potentially relevant in stereocilia considering that cofilin catalyses the disassembly of F-actin in filopodia [21] , which like stereocilia consists of parallel actin filaments crosslinked by fascin protein. In this study, we monitored actin dynamics by initiating irreversible expression of transgenic β-actin-green fluorescent protein (GFP) in adult mice and assessing its localization in stereocilia. We found that actin is remarkably stable in these structures, with slow incorporation of new β-actin-GFP monomers generally limited to stereocilia tips. In postnatal explants, the incorporation of β-actin-GFP at stereocilia tips was also slow, with a half-life of several hours. However, we observed that the stability of actin differed between the stereocilia in the tallest row of the bundle and those in the shorter rows. The shorter row stereocilia, which house mechanotransduction channels, incorporated higher levels of β-actin-GFP and showed marked variation among stereocilia. Severing may regulate actin turnover in these stereocilia because their lengths were improperly regulated in mice lacking ADF or expressing mutant AIP1. Altogether, these data demonstrate that F-actin cores of stereocilia shafts are exceptionally stable while also suggesting that actin filament severing is necessary for normal stereocilia length maintenance. Actin incorporation is limited to the distal tip compartment We previously detected rapid actin turnover in stereocilia only at the tips and not along the remainder of the stereocilia length [8] . Here we developed a novel system for assessing actin dynamics based on inducible β-actin-GFP expression. In this new system, transgenic β-actin-GFP expression is irreversibly initiated by the FLEx system [22] . Cre recombinase-mediated recombination removes an intervening tdTomato gene and flips the β-actin-GFP gene from the antisense to the sense orientation downstream of the chicken β-actin promoter. In transgenic mouse lines with constitutive, hair cell-specific Atoh1-Cre expression, β-actin-GFP expression was mosaic in inner hair cells (IHCs), outer hair cells (OHCs) and utricular hair cells ( Supplementary Fig. 1a–d ) [23] . To achieve conditional temporal control, we instead used a ubiquitously expressed tamoxifen-regulated CreER [8] . Following tamoxifen treatment, β-actin-GFP expression was induced in IHCs and utricular hair cells, but not in OHCs ( Supplementary Fig. 1e–j ). We compared the localization pattern of β-actin-GFP in IHC stereocilia 1, 2, 20 or 40 weeks after β-actin-GFP expression was initiated in adult (P21–25) mice by tamoxifen administration. In all cases, β-actin-GFP was detected within a small compartment at stereocilia tips and localization did not extend down the core of the stereocilia in row 1 of IHC bundles ( Fig. 1a–d ). To quantify the distribution of β-actin-GFP, we measured the GFP fluorescence intensity along lines extending from the tip of row 1 stereocilia towards the cell body. At all time points after β-actin-GFP expression started, fluorescence was observed as a peak localized within the first 0.5 μm from the tip ( Fig. 1e ). The intensity of β-actin-GFP fluorescence at stereocilia tips relative to background fluorescence increased between the 1-week, 2-week and 20-week time points, but remained constant between 20 and 40 weeks post-induction ( Fig. 1e ). Altogether, these results suggest that β-actin-GFP is slowly and continuously incorporated at stereocilia tips, reaching saturation between 2 and 20 weeks. Compared with that at stereocilia tips, β-actin-GFP was detected in stereocilia shafts to a lesser extent ( ∼ 1.5-fold over background compared with sevenfold at tips at 40 weeks; Fig. 1e ), with no clear increase in β-actin-GFP fluorescence with time following induction of expression. We conclude that β-actin-GFP is incorporated more rapidly and to a greater extent at stereocilia tips than in stereocilia cores. Furthermore, incorporation at the tip does not progress down the shaft as would be expected from an actin ‘treadmilling’ mechanism whereby actin filaments continuously polymerize at barbed ends within stereocilia tips, with concurrent depolymerization at the pointed ends at the stereocilia base. 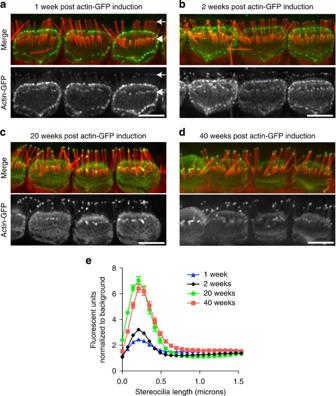Figure 1: β-Actin-GFP incorporation into mature IHC stereocilia is limited to a distal tip compartment. Transgenic β-actin-GFP expression was induced in mice at age P21–P25. Localization was assessed (a) 1 week, (b) 2 weeks, (c) 20 weeks or (d) 40 weeks after expression was initiated. β-Actin-GFP (green) localized to the tips of the tallest (row 1) stereocilia (arrow ina) and the tips of row 2 stereocilia (arrowhead ina), as well as to cell–cell contacts and the apical surface of the cell. F-actin is stained with phalloidin (red). (e) β-Actin-GFP fluorescence intensity was measured along the length of row 1 stereocilia from the tip towards the base and normalized to background fluorescence (n=76, 423, 118 and 134 stereocilia from at least three mice at 1, 2, 20 and 40 weeks, respectively. Error bars represent s.e.m.). Incorporation increased with time in the∼0.5-μm region at stereocilia tips, while remaining relatively constant in stereocilia shafts. Scale bars, 5 μm. Figure 1: β-Actin-GFP incorporation into mature IHC stereocilia is limited to a distal tip compartment. Transgenic β-actin-GFP expression was induced in mice at age P21–P25. Localization was assessed ( a ) 1 week, ( b ) 2 weeks, ( c ) 20 weeks or ( d ) 40 weeks after expression was initiated. β-Actin-GFP (green) localized to the tips of the tallest (row 1) stereocilia (arrow in a ) and the tips of row 2 stereocilia (arrowhead in a ), as well as to cell–cell contacts and the apical surface of the cell. F-actin is stained with phalloidin (red). ( e ) β-Actin-GFP fluorescence intensity was measured along the length of row 1 stereocilia from the tip towards the base and normalized to background fluorescence ( n =76, 423, 118 and 134 stereocilia from at least three mice at 1, 2, 20 and 40 weeks, respectively. Error bars represent s.e.m.). Incorporation increased with time in the ∼ 0.5-μm region at stereocilia tips, while remaining relatively constant in stereocilia shafts. Scale bars, 5 μm. Full size image Some stereocilia in shorter rows incorporate more actin Within IHC bundles, β-actin-GFP incorporation differed between stereocilia from the tallest row (row 1) and the shorter rows (rows 2 and 3). In row 1, β-actin-GFP incorporation was consistent among stereocilia, occupying a uniform zone of ∼ 0.5 μm and a uniform level, as gauged by GFP intensity ( Fig. 2a–i ; arrows). In contrast, β-actin-GFP incorporation in stereocilia in rows 2 and 3 was variable, with different intensities and distribution among stereocilia from the same IHC bundle ( Fig. 2a–i ; arrowheads). β-Actin-GFP incorporation was quantified by measuring GFP fluorescence intensity at row 1 stereocilia tips and row 2 or 3 stereocilia tips (which were not distinguished because they are of similar heights). The relative fluorescent intensities at tips and the distribution of intensities across stereocilia were compared by normalizing the value for each stereocilium with the row 1 average on a per cell basis ( Fig. 2j ). At each time point following induction of β-actin-GFP expression, fluorescent intensities for row 1 stereocilia were distributed over a narrow range, consistent with uniform β-actin-GFP incorporation across stereocilia. In contrast, rows 2 and 3 fluorescent intensities were distributed over a broader range and were up to fivefold higher than the row 1 average, and this trend increased with time after β-actin-GFP induction ( Fig. 2j ). 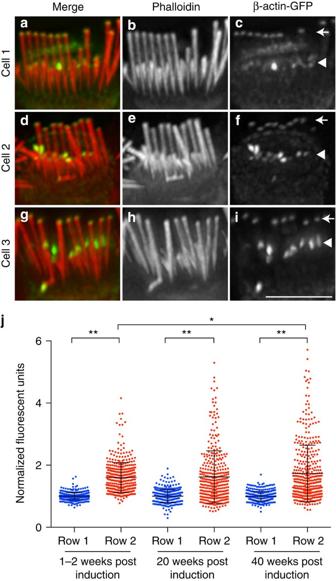Figure 2: Individual stereocilia in the shorter rows of bundles incorporate more actin. (a–i) Three examples of IHC stereocilia 20 weeks after β-actin-GFP expression was initiated. (a,d,g) Merged image of β-actin-GFP (green) and phalloidin (red); (b,e,h) phalloidin stain only; (c,f,i) β-actin-GFP only. Bundles showed varying levels of accumulation at the tips of the shorter row stereocilia (rows 2 and 3, arrowheads). In contrast, stereocilia in the tallest row (row 1, arrows) displayed very consistent levels of β-actin-GFP incorporation. (j) The fluorescence intensity of β-actin-GFP at the tips of row 2 and 3 stereocilia was compared with row 1 stereocilia at times 1–2 weeks, 20 weeks and 40 weeks after β-actin-GFP expression was initiated. Compared with row 1 stereocilia, row 2 and 3 stereocilia incorporated increased levels of β-actin-GFP with more variation between individual stereocilia. Fluorescence intensity was measured in at least 350 stereocilia per category from three or more mice. The mean is indicated with error bars representing s.d.; *P<0.01 and **P<0.001, analysis of variance. Scale bar, 5 μm. Figure 2: Individual stereocilia in the shorter rows of bundles incorporate more actin. ( a – i ) Three examples of IHC stereocilia 20 weeks after β-actin-GFP expression was initiated. ( a , d , g ) Merged image of β-actin-GFP (green) and phalloidin (red); ( b , e , h ) phalloidin stain only; ( c , f , i ) β-actin-GFP only. Bundles showed varying levels of accumulation at the tips of the shorter row stereocilia (rows 2 and 3, arrowheads). In contrast, stereocilia in the tallest row (row 1, arrows) displayed very consistent levels of β-actin-GFP incorporation. ( j ) The fluorescence intensity of β-actin-GFP at the tips of row 2 and 3 stereocilia was compared with row 1 stereocilia at times 1–2 weeks, 20 weeks and 40 weeks after β-actin-GFP expression was initiated. Compared with row 1 stereocilia, row 2 and 3 stereocilia incorporated increased levels of β-actin-GFP with more variation between individual stereocilia. Fluorescence intensity was measured in at least 350 stereocilia per category from three or more mice. The mean is indicated with error bars representing s.d. ; * P <0.01 and ** P <0.001, analysis of variance. Scale bar, 5 μm. Full size image Actin is stable in vestibular hair cell stereocilia We also assessed the localization of β-actin-GFP in utricular hair cells of the vestibular system. Utricular stereocilia, which detect head acceleration including gravitational force, are markedly longer than auditory hair cell stereocilia and are organized into more cylindrical bundles. As with IHC stereocilia, β-actin-GFP was detected at utricular stereocilia tips in the majority of cells as well as at the apex of the cell body 1 week after induction ( Fig. 3a,b ; white arrows). After 20 weeks of expression, this localization pattern persisted in the majority of cells, in which β-actin-GFP was only detected at stereocilia tips ( Fig. 3c,d ; white arrows). Intriguingly, we observed the occasional exception where β-actin-GFP was incorporated into a larger zone at the tips of a few stereocilia within a utricular hair cell bundle ( Fig. 3 ; blue arrowhead). As with IHC stereocilia, most stereocilia in the same bundle incorporated β-actin-GFP only at their tips, indicating that actin dynamics are independently regulated in individual stereocilia. Finally, we observed a third population of cells that had markedly shorter stereocilia, which were labelled with β-actin-GFP along their entire length ( Fig. 3c,d ; yellow arrows). These are likely nascent bundles that developed after β-actin-GFP expression was initiated. Indeed, live imaging of utricular hair cells demonstrates continuous incorporation of β-actin-GFP in elongating stereocilia [24] . Altogether, these data indicate that actin regulation is similar in vestibular and auditory stereocilia with both featuring very stable actin along the stereocilia length and limited actin incorporation at stereocilia tips. 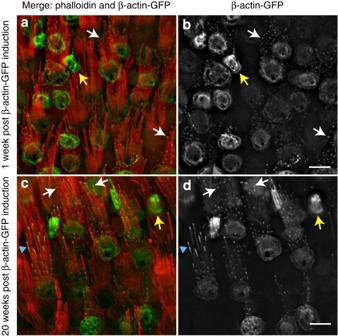Figure 3: Vestibular hair cell stereocilia incorporate actin only in the distal tip compartment. (a) One week. β-actin-GFP in green and F-actin stained with phalloidin in red. (b) Greyscale image of β-actin-GFP. β-Actin-GFP was incorporated in a small compartment at the tips of utricular hair cell stereocilia (examples indicated by white arrows). Yellow arrow indicates a cell that apparently lacked phalloidin-stained stereocilia but expressed β-actin-GFP. (c) Twenty weeks. β-Actin-GFP (green) and F-actin (red). (d) Greyscale image of β-actin-GFP. In most cells, β-actin-GFP incorporation remained restricted to stereocilia tips (examples indicated by white arrows). Other cells had a short bundle of stereocilia that contained β-actin-GFP along their length (yellow arrow), likely representing nascent bundles that developed in the 20 weeks following the start of β-actin-GFP expression. Occasionally, individual stereocilia in a bundle developed a longer zone containing β-actin-GFP (blue arrowhead), while other stereocilia in the same bundle had β-actin-GFP localization restricted to tips. Scale bar, 5 μm. Figure 3: Vestibular hair cell stereocilia incorporate actin only in the distal tip compartment. ( a ) One week. β-actin-GFP in green and F-actin stained with phalloidin in red. ( b ) Greyscale image of β-actin-GFP. β-Actin-GFP was incorporated in a small compartment at the tips of utricular hair cell stereocilia (examples indicated by white arrows). Yellow arrow indicates a cell that apparently lacked phalloidin-stained stereocilia but expressed β-actin-GFP. ( c ) Twenty weeks. β-Actin-GFP (green) and F-actin (red). ( d ) Greyscale image of β-actin-GFP. In most cells, β-actin-GFP incorporation remained restricted to stereocilia tips (examples indicated by white arrows). Other cells had a short bundle of stereocilia that contained β-actin-GFP along their length (yellow arrow), likely representing nascent bundles that developed in the 20 weeks following the start of β-actin-GFP expression. Occasionally, individual stereocilia in a bundle developed a longer zone containing β-actin-GFP (blue arrowhead), while other stereocilia in the same bundle had β-actin-GFP localization restricted to tips. Scale bar, 5 μm. Full size image Actin incorporation at stereocilia tips is slow To quantify actin dynamics at stereocilia tips, we measured β-actin-GFP fluorescence recovery after photobleaching in live IHC stereocilia. Organ of Corti explants were cultured from P6 mice constitutively expressing β-actin-GFP in hair cells, which enabled imaging of stereocilia in live cells by confocal microscopy. We photobleached rectangular regions of hair cell bundles and monitored fluorescence recovery by imaging the same cells at multiple time points. Within 75 min after bleaching, β-actin-GFP fluorescence was detectable at the tips of stereocilia, and these regions became more intense as recovery progressed ( Fig. 4a ). On the basis of the measurements from three-dimensional reconstructions, the zone of recovered β-actin-GFP in individual stereocilia of the same cells did not change in size between 400 min and 24 h after bleaching ( Supplementary Fig. 2 ). The drug cytochalasin D, which binds to the barbed ends of actin filaments and blocks polymerization [25] , decreased recovery at tips, indicating that recovery depends on the polymerization of new monomers at stereocilia tips ( Fig. 4b ). We quantified the fraction of fluorescence recovery at each time point by measuring the ratio of β-actin-GFP fluorescence in bleached spots to that at the tips of unbleached stereocilia in the same bundle ( Fig. 4c ). A single exponential curve was fitted and the calculated half-time of recovery was 215 min, which is markedly slower than actin assembly in solution, suggesting that filament ends are usually capped [26] . 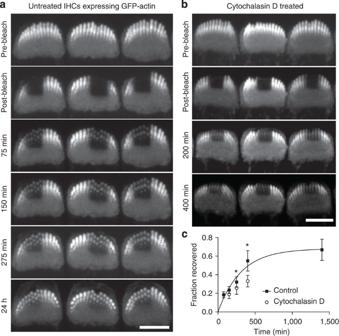Figure 4: β-Actin-GFP has a half-life of several hours at IHC stereocilia tips. Explants of organ of Corti from P6 mice constitutively expressing β-actin-GFP in hair cells were cultured for 48 h and live cells were imaged by confocal microscopy. (a) Rectangular regions of IHC stereocilia bundles were photobleached and recovery of β-actin-GFP was monitored in the same bleached cells for times up to 24 h post-bleaching. The tips of stereocilia recovered β-actin-GFP fluorescence over time. (b) Cytochalasin D, which prevents actin polymerization at filament barbed ends, slowed the recovery of β-actin-GFP fluorescence at stereocilia tips. (c) The ratio of β-actin-GFP fluorescence intensity at bleached stereocilia tips was compared with that of unbleached stereocilia tips (20 or more cells analysed per time point). The fraction recovered was plotted and fitted with a single exponential curve (T1/2=215 min). Error bars represent s.d., *P<0.01, analysis of variance. Scale bars, 5 μm. Figure 4: β-Actin-GFP has a half-life of several hours at IHC stereocilia tips. Explants of organ of Corti from P6 mice constitutively expressing β-actin-GFP in hair cells were cultured for 48 h and live cells were imaged by confocal microscopy. ( a ) Rectangular regions of IHC stereocilia bundles were photobleached and recovery of β-actin-GFP was monitored in the same bleached cells for times up to 24 h post-bleaching. The tips of stereocilia recovered β-actin-GFP fluorescence over time. ( b ) Cytochalasin D, which prevents actin polymerization at filament barbed ends, slowed the recovery of β-actin-GFP fluorescence at stereocilia tips. ( c ) The ratio of β-actin-GFP fluorescence intensity at bleached stereocilia tips was compared with that of unbleached stereocilia tips (20 or more cells analysed per time point). The fraction recovered was plotted and fitted with a single exponential curve ( T 1/2 =215 min). Error bars represent s.d., * P <0.01, analysis of variance. Scale bars, 5 μm. Full size image Actin severing is required for stereocilia maintenance β-actin-GFP incorporation at stereocilia tips must be balanced by actin disassembly since mature stereocilia lengths do not increase over time. Severing of actin filaments is a potential disassembly mechanism, and proteins that mediate filament severing—including ADF and AIP1—are detected in the chicken vestibular stereocilia proteome [9] . To determine whether the severing regulates stereocilia actin, we analysed hair cell morphology by scanning electron microscopy in mice either lacking ADF or bearing a mutant allele of Aip1 that results in reduced expression of AIP1 protein [27] . In control mice, both OHC and IHC stereocilia had normal morphology characterized by precise height registration of neighbouring stereocilia within a given row of the bundle ( Fig. 5a–c ). In contrast, rows 2 and 3 of OHC and IHC stereocilia bundles from both ADF knockout and mutant AIP1 mice were characterized by missing and shortened stereocilia ( Fig. 5d–k ). Stereocilia widths were modestly affected (156±22, 137±23 and 173±21 nm average±s.d. for control, AIP1 and ADF mutants, respectively, P <0.01, analysis of variance). Interestingly, the tallest (row 1) stereocilia appeared unaffected, with neighbouring stereocilia of similar heights present in normal numbers ( Fig. 5j,k ). These results show that changes in actin-severing dynamics directly impact rows 2 and 3 stereocilia length regulation. 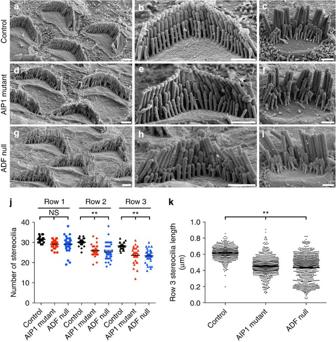Figure 5: ADF and AIP1 regulate the stereocilia morphology. (a–i) Scanning electron microscopy of control and mutant OHC and IHC stereocilia. (a–c) Control hair bundles. (d–f) AIP1 mutant. (g–i) ADF null. In each set, the left panel shows OHCs at lower magnification, the middle shows an OHC and the right shows an IHC at high magnification. AIP1 mutant and ADF null stereocilia in rows 2 and 3 were shorter, irregular in length or missing, while stereocilia in the tallest row were unaffected. Scale bars, 1 μm. (j) The number of stereocilia in rows 2 and 3 was reduced in OHCs from the AIP1 mutant and ADF null (20–30 cells from at least three mice). (k) OHC row 3 stereocilia from the AIP1 mutant and ADF null were shorter than control (500–800 stereocilia from at least three mice). (**P<0.001, analysis of variance). NS, not significant. Figure 5: ADF and AIP1 regulate the stereocilia morphology. ( a – i ) Scanning electron microscopy of control and mutant OHC and IHC stereocilia. ( a – c ) Control hair bundles. ( d – f ) AIP1 mutant. ( g – i ) ADF null. In each set, the left panel shows OHCs at lower magnification, the middle shows an OHC and the right shows an IHC at high magnification. AIP1 mutant and ADF null stereocilia in rows 2 and 3 were shorter, irregular in length or missing, while stereocilia in the tallest row were unaffected. Scale bars, 1 μm. ( j ) The number of stereocilia in rows 2 and 3 was reduced in OHCs from the AIP1 mutant and ADF null (20–30 cells from at least three mice). ( k ) OHC row 3 stereocilia from the AIP1 mutant and ADF null were shorter than control (500–800 stereocilia from at least three mice). (** P <0.001, analysis of variance). NS, not significant. Full size image Stereocilia length maintenance depends on regulation of the crosslinked bundle of actin filaments that form the stereocilia core. Multiple lines of evidence demonstrate that this core is exceptionally stable, perhaps reflecting the constant morphology and long-lived nature of stereocilia. In our earlier study, we measured slow protein turnover in stereocilia shafts compared with more rapid turnover at stereocilia tips using multi-imaging mass spectrometry [8] . Here we assessed actin incorporation in mature stereocilia in vivo by irreversibly initiating β-actin-GFP expression in adult hair cells. At multiple time points after induction, β-actin-GFP protein localized mainly in the distal tips of stereocilia, with very little incorporation in the shafts even after 40 weeks of β-actin-GFP expression. Although actin incorporation at stereocilia tips was markedly faster than in the core, the assembly rate measured by fluorescence recovery after photobleaching of β-actin-GFP in cultured explants was slow compared with that of pure actin in solution [26] , suggesting that abundant capping proteins found in stereocilia limit the availability of filament barbed ends [28] , [29] . A dynamic actin treadmill model previously proposed for stereocilia was based on the observations of transfected hair cell explants where β-actin-GFP was sometimes observed to extend from stereocilia tips partway down the shaft in fixed cells [30] , [31] . This localization pattern implied rapid and continuous actin incorporation at tips with concurrent depolymerization at the base to maintain a constant stereocilia length. However, time-lapse recordings from similar transfected explant preparations demonstrate that extended regions of β-actin-GFP incorporation correspond to stereocilia growth that occurs after the onset of β-actin-GFP expression, rather than incorporation into treadmilling filaments [24] . Stereocilia actin dynamics are thus markedly different from microvilli, where actin does treadmill, even though both structures are formed from parallel bundles of actin filaments [7] . Interestingly, exogenous espin-1, which is normally present in stereocilia tips, converts microvilli actin into a stable, non-treadmilling array, suggesting that it is part of a mechanism to stabilize actin in stereocilia [32] . Although stereocilia actin is generally stable, proper regulation, particularly at the tips, is essential for the maintenance of morphology. Loss of the crosslinking protein plastin-1 in mice results in tapered stereocilia tips and slowly progressive hearing loss, suggesting that plastin-1 crosslinks may limit actin barbed end depolymerization to prevent thinning of the actin bundle [33] . Mice lacking EPS8L2, a potential barbed end capping protein, develop a similar phenotype, although tapering of stereocilia tips is more pronounced in the shorter rows of stereocilia, likely reflecting the enrichment of EPS8L2 at their tips [34] . Finally, stereocilia tapering was also observed in developing and mature stereocilia of mice with reduced levels of the F-actin bundling protein espin [35] . Altogether, these data suggest that actin crosslinking stabilizes F-actin and prevents excessive actin turnover at stereocilia tips. Compared with the tallest row of stereocilia, we found that actin is more dynamic in individual stereocilia in the shorter rows of the hair cell bundle as demonstrated by their increased incorporation of β-actin-GFP ( Fig. 2 ). In the tallest row, the tagged actin accumulated strictly within a zone of ∼ 0.5 μm at stereocilia tips, and the intensity of β-actin-GFP fluorescence was very similar among all stereocilia in the row. In contrast, β-actin-GFP incorporation was more variable in the shorter rows of stereocilia, with some incorporating a significantly higher level of β-actin-GFP at their tips, and the zone of incorporation being larger, particularly at later time points. Therefore, actin turnover is apparently more dynamic at the tips of shorter row stereocilia. In addition, differential actin incorporation among shorter row stereocilia of a single cell suggests that actin is regulated at the level of individual stereocilia. The localization pattern of induced β-actin-GFP demonstrates that stereocilia actin cores are highly stable with a more dynamic zone at tips, but the dynamic tip zone is differentially regulated in the functionally distinct, shorter rows of stereocilia ( Fig. 6a ). 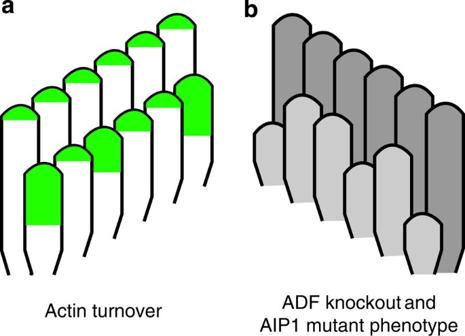Figure 6: Tip turnover model summarizing actin incorporation and regulation. (a) Green represents the regions where β-actin-GFP localized when expression was induced in mature auditory hair cells. The tallest row of stereocilia incorporated a uniform level of β-actin-GFP in each member of the row, while in shorter rows, some individual stereocilia incorporated markedly more β-actin-GFP. (b) Some individual stereocilia in the shorter rows of the bundle were shorter than their neighbours when hair cells lacked ADF or expressed mutant AIP1. We suggest a model in which individual stereocilia stochastically shorten and then require ADF and AIP1 to sever actin filaments, which exposes free barbed ends where new actin polymerization can drive regrowth. Figure 6: Tip turnover model summarizing actin incorporation and regulation. ( a ) Green represents the regions where β-actin-GFP localized when expression was induced in mature auditory hair cells. The tallest row of stereocilia incorporated a uniform level of β-actin-GFP in each member of the row, while in shorter rows, some individual stereocilia incorporated markedly more β-actin-GFP. ( b ) Some individual stereocilia in the shorter rows of the bundle were shorter than their neighbours when hair cells lacked ADF or expressed mutant AIP1. We suggest a model in which individual stereocilia stochastically shorten and then require ADF and AIP1 to sever actin filaments, which exposes free barbed ends where new actin polymerization can drive regrowth. Full size image Correspondingly, the shorter rows are particularly sensitive to perturbation of the actin cytoskeleton. Loss or mutation of several cytoskeletal proteins, including fascin-2 (ref. 36 ), β-actin [36] , Esp8L2 (ref. 34 ), AIP1 and ADF ( Fig. 5 ) results in a similar phenotype where some stereocilia in the shorter rows of the hair cell bundle shorten and lose precise height registration with their neighbours, while the tallest row remains more morphologically normal. The morphology of shorter row stereocilia is also uniquely regulated by tip links, which connect the tips of these stereocilia to the sides of those in the adjacent taller row. When tip links are lost, stereocilia in the tallest row are unaffected while stereocilia in the shorter rows remodel their tips, shorten and eventually disappear [38] , [39] , [40] . Altogether, these data suggest a model whereby individual stereocilia in the shorter rows of hair cell bundles shorten following stochastic tip link loss, with subsequent regrowth dependent on dynamic actin ( Fig. 6 ). Stereocilia from mice lacking ADF or expressing mutant AIP1 shortened ( Fig. 5 ). Since ADF/cofilin directly severs actin filaments, and its severing activity is potentiated by AIP1 (refs 10 , 12 , 13 , 14 ), it seems that severing normally stimulates stereocilia growth. In other cellular systems, filament severing promotes actin polymerization by generating new barbed ends, free of capping protein, where monomers can add [41] . Considering that stereocilia contain an abundance of capping proteins, which likely contribute to the stability of the actin core, a similar mechanism may promote actin assembly at stereocilia tips. Hair cell stereocilia adopt and maintain a specialized architecture that is required for their biological function. Here we demonstrate that the actin network in mature stereocilia is exceptionally stable with new actin incorporation occurring almost exclusively at stereocilia tips. Although stereocilia actin is largely static, dynamic behaviour at tips, regulated in part by actin severing, is required to maintain stereocilia lengths and preserve bundle morphology. Mouse lines The FLEx β-actin-GFP construct was generated by cloning mouse β-actin-EGFP sequence into a base FLEx vector [42] . The sequence elements are in the following order: chicken β-actin promoter/intron, lox2372, tdTomato and lox511 in the forward orientation, followed by β-actin-EGFP, lox2372 and lox511 in the reverse orientation before an SV40 polyA signal in the forward orientation. Linear, gel purified DNA was injected into C57BL/6 pronuclei, which were implanted into pseudopregnant mice by the Mouse Genetics Core at The Scripps Research Institute. Mice carrying the transgene were identified by PCR analysis of genomic DNA from tail snips. Myo7a::EGFP-β-actin, Atoh1-cre and Cagg-CreER lines were as previously described [8] , [37] . The Aip1 mutant is also known as Wdr1 rd and mice (Mouse Genome Informatics number MGI:2671870), generously provided by Monica Justice [27] , were backcrossed onto a C57BL/6 background. ADF null mice (also known as Dstn corn1/corn1 mice (B6.Cg-Dstn corn1 , MGI:1889311) were backcrossed onto a C57Bl/6 background [43] . Mouse lines were maintained using standard husbandry practices in AALAC accredited facilities. Institutional Animal Care and Use Committees of the University of Minnesota or Harvard Medical School approved all experimental procedures. Culture of explants Middle turns of the organ of Corti were dissected from mice at the indicated postnatal day in DMEM/F12 (Invitrogen, Carlsbad, CA, USA; catalogue number 11039) and adhered to a coverslip coated with Matrigel (BD Biosciences, San Jose, CA, USA; catalogue number 356230) for 2 h at 37 °C. Media was then exchanged for culture media consisting of DMEM (Invitrogen; catalogue number 10569) supplemented with 7% foetal bovine serum and 1 μg ml −1 ampicillin and explants were cultured at 5% CO 2 and 37 °C. Samples were transferred to room temperature dissection media for imaging and returned to culture media as above between time points. Imaging For fixed samples, anesthetized mice of the indicated age and genotype were killed by cervical dislocation and decapitated. Cochleae were dissected, the round and oval window membranes were removed and a hole was made in the apex before the tissue was fixed for 4 h at room temperature in 4% paraformaldehyde in PBS. Tissue was rinsed in PBS, and decalcified in 170 mM EDTA in PBS for 16 h at 4 °C. The organ of Corti and utricle were dissected, permeabilized in 0.2% Triton X-100 and stained with phalloidin conjugated to either Alexa-568 or Alexa-660 (Invitrogen). Samples were mounted in ProLong Antifade Reagent (Invitrogen) and imaged using an Applied Precision DeltaVision Deconvolution Microscopy system with either a × 100 numerical aperture (NA) 1.40 or × 40 NA 1.35 objective. β-Actin-GFP in live cultures was imaged by a confocal microscopy with a 488-nm laser using an upright Olympus FluoView 1,000 with a × 60 NA 1.1 water immersion objective. Regions of hair cell stereocilia bundles were bleached using a 405-nm laser. The calculated resolution of this system is 0.215 μm in X–Y and 1.16 μm in Z. To quantify fluorescence recovery, the tips of stereocilia were identified by scrolling through the stack of confocal images and integrated density was measured in a circular region of interest from a single plane using ImageJ software. Regions of identical size were measured from both bleached and unbleached stereocilia from the same bundle, the average value for each region was calculated for each hair cell at each time point, and the bleached value was divided by the unbleached value to determine the fraction recovered. Scanning electron microscopy Cochleae were dissected from mice. After removing the round and oval window membranes and making a small hole in the apex, the tissue was fixed by immersing in a solution of 2.5% glutaraldehyde, 1 mM CaCl 2 and 0.1 M sodium cacodylate for 4 h at room temperature before decalcification in 170 mM EDTA at 4 °C for 16 h. The organ of Corti was dissected and successively incubated in 2% each arginine, glycine, glutamic acid and sucrose in water, 2% each tannic acid and guanidine-HCl in water and then 1% osmium tetroxide. Samples were transitioned to ethanol, critical point dried from CO 2 and sputter coated with gold before viewing on a Hitachi S4700 field emission scanning electron microscope. Length measurements were made using ImageJ software. How to cite this article : Narayanan, P. et al . Length regulation of mechanosensitive stereocilia depends on very slow actin dynamics and filament-severing proteins. Nat. Commun . 6:6855 doi: 10.1038/ncomms7855 (2015).